Cationic-palladium catalyzed regio- and stereoselectivesyn-1,2-dicarbofunctionalization of unsymmetrical internal alkynes 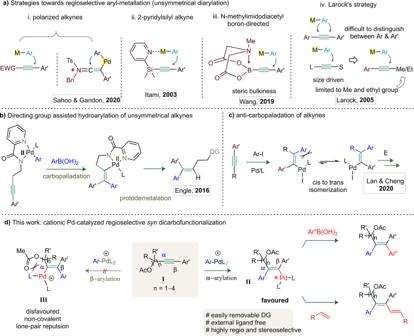Fig. 1: Comparison between hydro- and difunctionalization of alkynes and the conceptual blueprint of a general cationic Pd-catalyzed dicarbofunctionalization of Yne-acetates. a(i) Difunctionalization of electronically polarized alkynes: the incoming aryl group forms bond at the electron-deficient carbon center. (ii) Difunctionalization of 2-pyridylsilyl alkynes: the metal coordination to the pyridyl-N makes the C-aryl bond β to silyl group. (iii) Difunctionalization of N-methylimidodiacyl boron alkynes: the aryl group approaches the less-hindered side of borylated-alkyne. (iv)syn-1,2-Diarylation of diaryl-substituted alkynes occurs at an elevated temperature, providing a mixture of regioisomers. In case of aryl-alkyl alkynes, only the smaller alkyl groups (i.e., methyl/ethyl) allow the aryl-moiety to approach from the less-hindered side of the alkyne.bPd-catalyzed aminopyridine-directed regioselective hydroarylation of alkynes happens through proximity-driven carbopalladation followed by protodemetalation.canti-carbopalladation of alkyne driven by steric repulsion betweenortho-substituted aryl halide and bulky-ligands.dOur strategy: regioselective dicarbofunctionalization of yne-acetates: because of the non-covalent lone pair repulsion between ligated Pd and the carbonyl of acetate group, the ligated cationic Pd species preferably approaches at the β -carbon over α-carbon of the yne-acetate; as a result, intermediateIIis favored over intermediateIII. π-Extended tetrasubstituted olefins are widely found motifs in natural products, leading drugs, and agrochemicals. Thus, development of modular strategies for the synthesis of complex all-carbon-substituted olefins always draws attention. The difunctionalization of unsymmetrical alkynes is an attractive approach but it has remained faced with regioselectivity issues. Here we report the discovery of a regio- and stereoselective syn -1,2-dicarbofunctionalization of unsymmetrical internal alkynes. A cationic Pd-catalyzed three-component coupling of aryl diazonium salts, aryl boronic acids (or olefins) and yne-acetates enables access to all-carbon substituted unsymmetrical olefins. The transformation features broad scope with labile functional group tolerance, building broad chemical space of structural diversity (94 molecules). The value of this synthetic method is demonstrated by the direct transformation of natural products and drug candidates containing yne-acetates, to enable highly substituted structurally complex allyl acetate analogues of biologically important compounds. Synthetic versatility of the carboxylate bearing highly substituted olefins is also presented. The reaction outcome is attributed to the in situ formation of stabilized cationic aryl-Pd species, which regulates regioselective aryl-palladation of unsymmetrical yne-acetates. Control experiments reveal the synergy between the carboxylate protecting group and the cationic Pd-intermediate in the regioselectivity and reaction productivity; density functional theory (DFT) studies rationalize the selectivity of the reaction. Tetrasubstituted and π-extended olefins are widespread in numerous natural products, leading drugs, and agrochemicals. They also hold potential applications in electron-transport materials and light-emitting diodes [1] , [2] , [3] , [4] . The carbometallation of unsaturated C–C bonds has always been a gateway to biologically valuable feedstocks. In this regard, the carbopalladation has been the most prominent and widely used process [5] . The transition metal-catalyzed alkyne dicarbofunctionalization by interrupting two cross-couplings [for example: Suzuki and Heck] offers a potential entry to highly substituted olefins. However, in contrast with the directed olefin dicarbofunctionalization [5] , [6] , [7] , [8] , [9] , [10] , [11] , [12] , [13] , [14] , this approach often suffers from insolvable regioselectivity issues. Mostly, the state-of-the-art regioselective carbometallation of unsymmetrical alkynes is restricted to inherently polarized substrates (Fig. 1a-i ) [15] , [16] , [17] , [18] , [19] , [20] , [21] , [22] , [23] , [24] , [25] , [26] , [27] , [28] , [29] , [30] , 2-pyridylsilyl alkynes (Itami; Fig. 1a-ii ) [31] , [32] , [33] or sterically hindered borylated alkynes (Wang; Fig. 1a-iii ) [34] . The Larock’s Pd-catalyzed syn -1,2-diarylation of unsymmetrical alkynes is also a great strategy to access all-carbon-substituted olefins (Fig. 1a-iv ); however, it suffers from several limitations [35] , [36] . For instance, syn -1,2-diarylation of diaryl-substituted alkynes occurs at an elevated temperature to deliver a mixture of regioisomers in moderate selectivity (Fig. 1a-iv ). In case of aryl-alkyl alkynes, the arylation takes place at the less-hindered site of alkyne, resulting in better regioselectivity (Fig. 1a-iv ), but only with Me and Et groups. Thus, the syn -1,2-diarylation of unsymmetrical alkynes is substrate specific. An interesting aminopyridine directing group (DG) guided regioselective hydroarylation of alkynes with aryl boronic acids for the construction of trisubstituted olefins has also been described (Engle, Fig. 1b ) [37] , [38] . Overall, DG, ligand and the electron-bias of the alkyne are essential features in regioselective alkyne difunctionalization. The recent reports of Lan and Cheng feature an impressive DG free anti -carbopalladation of internal alkynes, the steric clash between the ortho -substituted aryl halide and the bulky ligated Pd(II) species making the anti-addition to alkyne possible at an elevated temperature [39] . In addition, Werz and co-workers designed an anti -carbopalladation reaction within a cascade process via 14 valence electron Pd species as crucial intermediates [40] , [41] , [42] . In this context, the development of a ligand free regioselective syn-1,2-dicarbofunctionalization of unsymmetrical alkynes to build tetrasubstituted olefins appears to be a worthwhile endeavor. 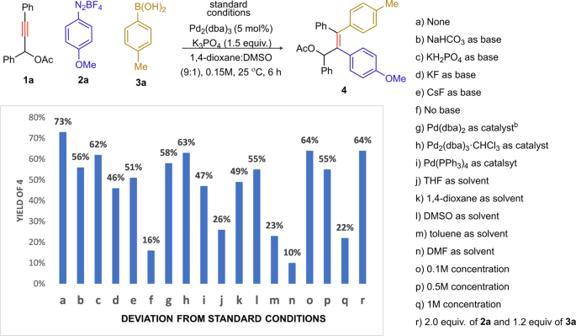Fig. 2: Optimization of the reaction conditionsa. aIsolated yield. 1a (0.2 mmol), 2a (0.6 mmol), 3a (0.3 mmol), cat. (0.01 mmol) and base (0.45 mmol).b10 mol%. Fig. 1: Comparison between hydro- and difunctionalization of alkynes and the conceptual blueprint of a general cationic Pd-catalyzed dicarbofunctionalization of Yne-acetates. a (i) Difunctionalization of electronically polarized alkynes: the incoming aryl group forms bond at the electron-deficient carbon center. (ii) Difunctionalization of 2-pyridylsilyl alkynes: the metal coordination to the pyridyl-N makes the C-aryl bond β to silyl group. (iii) Difunctionalization of N-methylimidodiacyl boron alkynes: the aryl group approaches the less-hindered side of borylated-alkyne. (iv) syn -1,2-Diarylation of diaryl-substituted alkynes occurs at an elevated temperature, providing a mixture of regioisomers. In case of aryl-alkyl alkynes, only the smaller alkyl groups (i.e., methyl/ethyl) allow the aryl-moiety to approach from the less-hindered side of the alkyne. b Pd-catalyzed aminopyridine-directed regioselective hydroarylation of alkynes happens through proximity-driven carbopalladation followed by protodemetalation. c anti -carbopalladation of alkyne driven by steric repulsion between ortho -substituted aryl halide and bulky-ligands. d Our strategy: regioselective dicarbofunctionalization of yne-acetates: because of the non-covalent lone pair repulsion between ligated Pd and the carbonyl of acetate group, the ligated cationic Pd species preferably approaches at the β -carbon over α-carbon of the yne-acetate; as a result, intermediate II is favored over intermediate III . Full size image We herein report a cationic Pd-catalyzed 1,2-dicarbofunctionalization of unsymmetrical alkynes (Fig. 1c ). As per DFT studies (vide infra), the reaction relies on a site-selective coordination of a cationic Pd(II) species, generated in situ by the oxidative addition of an aryl diazonium salt [43] , [44] to Pd(0), to an yne-acetate ( I ) (Fig. 1c ). This results in a syn -α-arylated-Pd-intermediate II . The lone pair repulsion between the carboxylate moiety and the Pd-complex possibly excludes syn -β-arylated-Pd-intermediate III . Further functionalization of vinyl-Pd(II)-cationic species II with aryl boronic acids (or olefins) delivers highly substituted olefins (or dienes). This strategy leads to structurally diverse all-carbon-functionalized olefins (94 molecules) in a single step from readily available yne-acetates. The transformation is highly regio- and stereoselective, even in the absence of external ligand and DG. A comparativereactivity profile and mechanistic pathway of the current method over Larock’s strategy for high regioselectivity throughput is established by various control experiments. Reaction optimization To investigate the 1,2-diarylation of structurally simple yne-acetates [i.e. propargyl acetates (PAs) to start with], a three-component reaction of 1,3-diphenylprop-2-yn-1-yl acetate ( 1a ), p –methoxyphenyl diazonium tetrafluoroborate ( 2a ), and p –tolyl boronic acid ( 3a ) in presence of Pd 2 (dba) 3 as the catalyst and a base was performed (Fig. 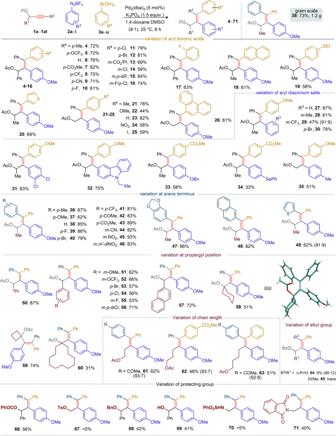Fig. 3: Scope of alkynes, aryl boronic acids, and aryl diazonium saltsa. All yields correspond to products isolated as a single stereo- and regioisomer, unless otherwise stated.a1(0.3 mmol),2(0.9 mmol),3(0.45 mmol). Ac acetyl and Bz benzyol. 2 ; see also Supplementary Table 3 , SI). An extensive screening led to the optimized reaction conditions: [ 1a (1.0 equiv), 2a (3.0 equiv), 3a (1.5 equiv), Pd 2 (dba) 3 (5.0 mol%) and K 3 PO 4 (1.5 equiv) in 1,4-dioxane/DMSO (9:1) at 25 °C, 6 h]. With these, the unsymmetrical syn -diarylation product 4 was isolated in 73% yield (Fig. 2 , a ). NaHCO 3 , KH 2 PO 4 , KF and CsF proved to be less efficient bases ( b – e ). Compound 4 was isolated in 16% in the absence of base ( f ). Lower yields were obtained when other Pd(0) catalysts [Pd(dba) 2 , Pd 2 (dba) 3 . CHCl 3 , Pd(PPh 3 ) 4 ,] were used ( g – i ). The solvents THF, 1,4-dioxane, DMSO, toluene or DMF did not improve the outcome ( j – n ). The reaction concentration did influence the product yield 4 ( o – q ). The reaction was less efficient when 2a (2.0 equiv) and 3a (1.2 equiv) were used ( r ). Fig. 2: Optimization of the reaction conditions a . a Isolated yield. 1a (0.2 mmol), 2a (0.6 mmol), 3a (0.3 mmol), cat. (0.01 mmol) and base (0.45 mmol). b 10 mol%. Full size image Scope of unsymmetrical diarylation This breakthrough encouraged us to investigate the reaction scope (Figs. 3 – 5 ). The reactivity of the aryl boronic acid partners was first probed (Fig. 3 ). The reaction of electron-rich p -substituted aryl boronic acids [ p -Me ( 3a ), p -OCF 3 ( 3b )] with 1a and 2a provided 4 and 5 in good yields. Likewise, the tetrasubstituted olefins 6 – 9 (62–76 %) were constructed from phenylboronic acid ( 3c ) and electron-poor aryl boronic acids [ p -CO 2 Me ( 3d ), p -CF 3 ( 3e ), p -CN ( 3f )] when exposed to 1a and 2a . Although halo groups are usually amenable to cross-couplings under Pd(0)-catalysis, to our delight, the halogen-substituted aryl boronic acids [ p -F ( 3g ), p -Cl ( 3h ), p -Br ( 3i )] proved compatible with the title reaction, leading to 10 – 12 in good yields. The transformation was compatible with meta - and ortho -substituted aryl boronic acids as well, leading to the densely functionalized tetrasubstituted olefins 13 – 17 (59–84%). The desired 2-naphthyl, 4-ethylthiophenyl, 3-thienyl-bearing allyl acetates 18 – 20 (58–69%) were also assembled from the methyl-substituted yne-acetate 1b . The unsubstituted PA 1c also proved to be a relevant substrate; various aryl boronic acids [ p -Me ( 3a ), p -OMe ( 3r ), p -H ( 3c ), p -NO 2 ( 3s ), and p -I ( 3t )] were coupled to provide 21 – 25 . The bulky 9-phenanthrene boronic acid was not an exception, providing the π-extended product 26 in 61% yield. Next, the three-component couplings of aryl diazonium tetrafluoroborates 2 with 1b and 3r / 3d were surveyed. The reaction of 1b , 3r and diverse arene diazonium salts [phenyl ( 2b ), electron-rich m -Me ( 2c ), electron-poor m -CF 3 ( 2d ), p -Br ( 2e ), and m , p -diCl ( 2f )] provided 27 – 31 in good yields. The allyl acetate 29 was isolated as regioisomeric mixture (91:9). A carbazole bearing diarylation product 32 was isolated in 75% yield. The OBn protecting group and the oxidizable SePh group were unaffected under this Pd-catalysis, giving access to 33 and 34 . Likewise, 35 (51%) was made from the reaction of 1c with 2j and 3r . We next scrutinized the reactivity of unsymmetrical alkynes (Fig. 3 ). The reaction of PAs [having aryl motifs: p ‐Me, p -OMe, p ‐F, p -Br, p -CF 3 , p -COMe, p -CO 2 Me, m -CN, m ‐NO 2 , m,m ′-diNO 2 , and m,p ‐methylenedioxy at the alkyne terminus] with 2a and 3c independently furnished the desired products 36 – 47 (62–93%). Likewise, the π-extended 2-naphthyl- and heteroaryl 2-thienyl-enabled tetrasubstituted olefins 48 and 49 were constructed. Irrespective of n -propyl and various aryl-moieties at the propargyl position of PAs, the diarylation was equally effective in making 50 – 57 . In general, sterically bulky substituents severely affect cross-couplings. Nevertheless, syn -diarylation of cyclohexyl and cyclobutyl tethered PAs with 2a and 3c provided all-carbon-substituted olefins 58 and 59 . X-ray analysis confirmed the structure of 58 (CCDC 2096145 contains the supplementary crystallographic data for compound 58). A macrocycle dodecane tethered diarylation product 60 was also fabricated. However, the terminal ynamide led to a complex mixture instead of providing the respective diarylation product. The product complexity justifies moderate yields (<50%); in such cases, the reaction was incomplete with recovery of unreacted PAs. To test the potential coordination ability of the carboxylate group, diarylation of yne-acetates with different tether lengths between the alkyne and the acetate functionalities was probed. Irrespective of the acetate position in yne-acetates, syn -diarylation of alkyne motifs was highly regioselective, furnishing 61 – 63 in moderate yields (Fig. 3 ). The diarylation of alkyl-substituted PAs 1ae / 1af independently with 2a and 3c under the optimized condition has led to 64 ( 9%) and 65 (trace). In these cases, reaction was complex forming arylative dimerization of alkyne (confirmed by HRMS analysis) along with unreacted precursors (see the SI Supplementary Figs. 19 and 32 ). Next, the reaction of O-benzoate and O-benzyl protected propargyl alcohols with 2a and 3c afforded 66 (56%) and 68 (42%) respectively. On the other hand, the reaction of O-tosyl protected alkyne led to a complex mixture including a low amount of 67 (<5%); the low yield is possibly due to the facile cleavage of the labile C–OTs bond. The reaction of alkynes having unprotected hydroxy group or phthalimide group at the propargyl position with 2a and 3c delivered the desired diarylation products 69 and 71 in moderate yield with good regioselectivity. Unfortunately, the identical transformation of propargyl sulfonamide did not give the desired diarylation product 70 . The reaction is scalable to the gram, as shown by the preparation of 38 (1.2 g, 73 %) from the coupling of 1a (1.0 g, 2.67 mmol), 2a (1.77 g, 8.01 mmol) and 3c (0.5 g, 4.00 mmol) using Pd 2 (dba) 3 (3.0 mol %) (Fig. 3 ). Fig. 3: Scope of alkynes, aryl boronic acids, and aryl diazonium salts a . All yields correspond to products isolated as a single stereo- and regioisomer, unless otherwise stated. a 1 (0.3 mmol), 2 (0.9 mmol), 3 (0.45 mmol). Ac acetyl and Bz benzyol. Full size image Fig. 4: Scope of aryl-olefination of alkynes a . All yields correspond to products isolated as a single stereo- and regioisomer, unless otherwise stated. a 1 (0.3 mmol), 2 (0.9 mmol), 72 (0.45 mmol). a Hydroarylation product was observed (see 117 , Fig. 6d ). ND not determined. Full size image Fig. 5: Scope of diarylation of biologically relevant motif coupled alkynes and synthetic applications. All reactions are carried out on a 0.2 mmol scale. All the compounds are isolated as a single isomer, unless otherwise stated. P -TSA p -tolylsulfonic acid, DMP Dess–Martin periodinane. Full size image Substrate scope of aryl-alkenylation π-Conjugated scaffolds are widely found in molecules of pharmaceutical importance and light-emitting-diode materials [1] . We thus attempted to trap the cationic vinyl palladium species, obtained after aryl-palladation of the alkyne moiety, with olefins for constructing π-conjugated dienes (Fig. 4 ). As envisaged, the reaction of 1b , 2a and ethyl acrylate ( 72a ) under the optimized conditions of entry 1, Fig. 2 , successfully led to 73 in 66% yield. 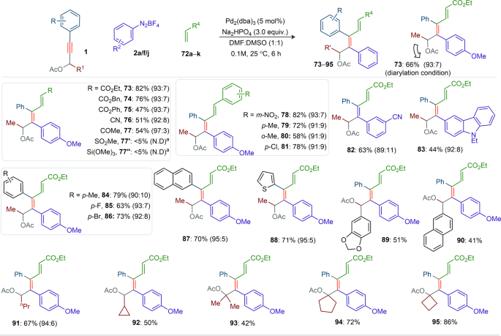Fig. 4: Scope of aryl-olefination of alkynesa. All yields correspond to products isolated as a single stereo- and regioisomer, unless otherwise stated.a1(0.3 mmol),2(0.9 mmol),72(0.45 mmol).aHydroarylation product was observed (see117, Fig.6d). ND not determined. To enhance the reaction productivity, bases and solvents were further screened (Supplementary Table 4 , SI). The Na 2 HPO 4 base and DMSO:DMF (1:1) solvent combination were found optimum; 73 was isolated in 82% yield. Next, the reaction of wide ranges of acrylates and acrylonitriles with 1b and 2a under the adapted catalytic conditions furnished the desired conjugated dienes such as 73 (82%, 93:7), 74 (76%, 93:7), 75 (47%, 93:7) and 76 (51%, 92:8). Methyl-vinyl ketone is usually susceptible to polymerization [45] ; despite this potential issue, 77 was isolated in 54% yield and 97:3 regioisomeric ratio. This difunctionalization even worked with styrenes, affording 78 (93:7), 79 (91:9), 80 (91:9), and 81 (91:9) in 58–82% yield. However, identical transformations with methyl-vinyl sulfone or vinyltrimethoxysilane did not provide the desired aryl-alkenylation products 77′ and 77″ . Rather substantial amount of hydroarylation product was observed along with unreacted yne-acetate. The products 82 (63%, 89:11) and 83 (44%, 92:8) were made from the couplings of 1b and 72a with 2f and 2j , respectively. The PAs [having aryl motifs: p -Me, p -F, p -Br, π-extended 2-naphthyl or 2-thienyl at the alkyne terminus] were independently coupled with 2a and 72a to deliver 84 – 88 in good yields along with 5–10% minor isomer. Likewise, 89 – 91 were made, albeit in moderate yield, from the reaction of PAs [with variation of substituents, m,p -methylenedioxy-phenyl, 2-naphthyl, n -Pr, and cyclopropyl at the propargyl position] with 2a and 72a . Even the sterically encumbered di-Me, cyclopentyl, and cyclobutyl tethered PAs were successfully converted into unusual π-conjugated dienes 92 – 95 (42–86%). Thus, the cationic Pd-catalytic system did not virtually affect the reaction outcome and the strained cyclopropyl ring, labile halo groups, and easily modifiable functional groups were well tolerated (Figs. 3 and 4 ). Scope of pharmacophore-coupled alkynes and synthetic applications Late-stage difunctionalization of unsymmetrical alkynes having biologically relevant motifs (BRMs) is invaluable for the sustainable development of complex molecules with enhanced pharmacokinetic properties. However, BRMs with polar groups and unsaturated moieties often cause problems for cross-coupling reactions, as the TM binding ability could lead to substrate decomposition and affect the difunctionalization efficiency. We were therefore intrigued by the viability of the cationic Pd-catalyzed double arylation of pharmacophore-coupled alkynes 1 (Fig. 5 ). Once again, the title reaction proved reliable: tetrasubstituted allyl acetates encapsulated fatty alcohol [vitamin-E-tocopherol ( 96 )], steroid [cholesterol ( 97 )], and terpenoid [geraniol ( 98 )] were produced in 45–72% yields from the diarylation of respective BRMs-coupled PAs with 2a and 3c . We further probed the efficacy of the regioselective diarylation using marketed drug molecules containing unsymmetrical alkynes. Thus, reaction of the anti-epileptic drug, bipolar disorder, and migraine preventer valproic acid coupled PA with 2a and 3c provided highly substituted allyl acetate 99 in 65% yield. Likewise, nonsteroidal anti-inflammatory drug containing allyl acetate 100 was made in good yield. We next probed the synthetic versatility of the newly constructed tetrasubstituted allyl-acetates. The p ‐TSA driven intramolecular Friedel-Crafts arene cyclization of 58 / 59 led to unusual cyclohexyl/cyclobutyl spiro-fused indene derivatives 101 (65%) and 102 (83%), respectively, and peripheral-substituted indenes 38 \({{\to }}\) 103 (89%) and 4 \({{\to }}\) 104 (79%). Likewise, electrophilic cyclization of 23 provided indanone 105 in 58% yield. Fully substituted propargyl alcohols [ 38 \(\to\) 106 (81%); 23 \({{\to }}\) 1 07 (77%)] were accessed from the KOH mediated hydrolysis of the acetate motif. Dess–Martin periodinane (DMP)-mediated oxidation of 106 and 107 delivered methyl-vinyl ketone 108 (78%) and acrolein 109 (72%), respectively; further functionalization of carbonyl groups is therefore possible. Allylation and hydrolysis of π-extended ester 73 yielded allylic-3°-alcohol 110 and α,β-unsaturated carboxylic acid 111 . Mechanistic studies To shed light on the reaction mechanism and importance of ArN 2 BF 4 , cationic palladium species, and acetate (OAc) group for the notable regioselectivity outcome in the 1,2-diarylation of PAs, a series of experiments was planned (Fig. 6a–d ). The reaction of electronically diverse PAs (having aryl-moiety p -OMe ( 1au )/ p -COMe ( 1av ) at the alkyne terminus) were independently subjected to different reaction conditions: {Larock’s conditions: eq 1 [ p -methoxyphenyl (PMP)-I, PhB(OH) 2 , Pd(PhCN) 2 Cl 2 , K 2 CO 3 , DMF:H 2 O (4:1), rt]}, {standard conditions (SC) of current reaction: eq 2 [PMP-N 2 BF 4 , PhB(OH) 2 , Pd 2 (dba) 3 , K 3 PO 4 , 1,4-dioxane:DMSO (9:1), rt]}, and {SC of current reaction: eq 3 [PMP-I instead PMP-N 2 BF 4 ]}. As anticipated, the diarylation products 112 (57%) and 113 (74%) with regioisomeric excess ( re ) 100% and 94%, respectively, were formed (eq 2, Fig. 6a ). On the other hand, the identical reaction under Larock’s conditions provided poor productivity as well as low re 112 (11%, 50% re ) and 113 (21%, 56% re ) (eq 1, Fig. 6a ). In comparison, 112 (13%, 54% re ) and 113 (24%, 20% re ) were observed when the reaction was performed with PMP-I instead PMP-N 2 BF 4 under the SC (eq 3, Fig. 6a ). It appears that cationic palladium species [obtained in situ by the oxidative addition of PMP-N 2 BF 4 with Pd(0) catalyst] play a crucial role in the control of the regioselectivity as well as productivity. Likewise, 1,2-diarylation of p -MeO-C 6 H 4 ( 1aw )/ p -MeOC-C 6 H 4 ( 1ax )- n butyl alkynes with PMP-I/ PMP-N 2 BF 4 along with PhB(OH) 2 independently led to [ 114 (38%, 68% re ) and 115 (42%, 82% re ) under Larock’s conditions, shown in eq 4, Fig. 6b ] and [ 114 (61%, 78% re ) and 115 (70%, 80% re ) under SC, shown in eq 5, Fig. 6b ]. Thus, 114 (~70% re ) and 115 (~80% re ) with regioisomeric products mixture obtained in the diarylation of 1ar / 1as (with no carboxylate moiety) irrespective of Larock/SC suggests that alkynes with electronic variation marginally affect both selectivity and productivity. On the other hand, diarylation of yne-acetates occurs with excellent regioselectivity (eq 2, Fig. 6a ); notably, the electronic properties of functional groups did virtually not show any impact. Fig. 6: Mechanistic studies. 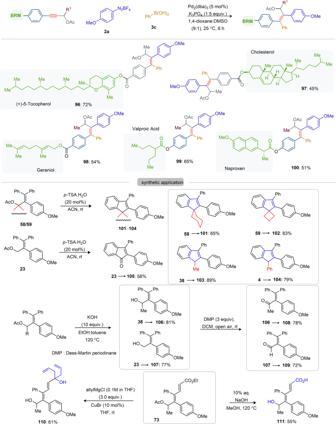Fig. 5: Scope of diarylation of biologically relevant motif coupled alkynes and synthetic applications. All reactions are carried out on a 0.2 mmol scale. All the compounds are isolated as a single isomer, unless otherwise stated.P-TSAp-tolylsulfonic acid, DMP Dess–Martin periodinane. a Three comparative reactions were performed with electronically diverse propargyl acetates under the {Larock’s reaction conditions: eq 1 [PMP-I, PhB(OH) 2 , Pd(PhCN) 2 Cl 2 , K 2 CO 3 , DMF:H 2 O (4:1), rt]}, {standard conditions (SC) of current reaction: eq 2 [PMP-N 2 BF 4 , PhB(OH) 2 , Pd 2 (dba) 3 , K 3 PO 4 , 1,4-dioxane:DMSO (9:1), rt]}, and {SC of current reaction: eq 3 [PMP-I instead of PMP-N 2 BF 4 ]}. Excellent regioselectivity has been observed in eq 2; thus, PMP-N 2 BF 4 and cationic palladium species are pivotal. b Two comparative reactions were performed with electronically diverse aryl-butyl alkynes using Larock’s reaction conditions (eq 4) and the SC of current reaction (eq 5). c Two comparative reactions were independently performed with sterically hindered Ph-cyclohexyl alkyne and cyclohexyl tethered PA under the Larock’s reaction conditions (eqs. 6 and 8) and SC current reaction (eq. 7), respectively. d Trapping of cationic vinylic Pd(II) species in the absence of aryl boronic acid. Note: inseparable regioisomers are isolated as mixture and the regioisomeric excess (re) is determined by 1 H NMR. PMP p -methoxyphenyl. Full size image To further validate the importance of the acetate group, sterically hindered phenyl cyclohexyl alkyne 1ay was subjected to PMP-I, and PhB(OH) 2 under Larock’s reaction conditions (eq. 6, Fig. 6c ); the respective product 116 (28%, 74% re ) was isolated in low yield and moderate regioselectivity (eq 6, Fig. 6c ). By contrast, reaction of 1y , exhibiting an acetate group at the propargyl position of 1ay , with PMP-N 2 BF 4 and PhB(OH) 2 under the SC furnished 58 (51%) in 100% re (eq 7, Fig. 6c ). Moreover, 1y failed to give the desired diarylation product 58 under Larock condition, thus, cationic Pd species is essential (eq 8, Fig. 6c ). From the mechanistic discussions highlighted in eqs 1–8, Fig. 6 , we conclude that the outcome and regioselectivity of syn -1,2-diarylation of unsymmetrical alkynes are strongly influenced by the carboxylate protecting group and the in situ formation of a stabilized cationic Pd intermediate. DFT calculations To gain insight into the reaction mechanism and notably the stereo/regioselectivity of the 1,2-diarylation of PAs, DFT calculations were performed at the M06L/def2-TZVPP(SMD)//BP86/LANL2DZ(Pd)_6-31G(d,p) level of theory (Fig. 7 , see also the SI for the cross-coupling part, the case of substrates with longer tethers and the case of an unreactive methylalkyne). The transformation begins with the barrierless oxidative addition of Pd(DMSO) 2 ( a ) to the phenyl diazonium salt b to provide the cationic Pd-complex 1 A . 6a Next, coordination of 1 A to PA 1c is possible by substitution of N 2 . However, this process could happen in three different ways, via (i) the coordination of the C≡C bond of 1c to form complex 1 B by releasing 6.7 kcal/mol of free energy (Fig. 7 ; blue) (ii) the coordination of both the C≡C bond and the ester group in 1c to provide 1 E with the release of 4.5 kcal/mol of free energy (Fig. 7 ; red), and (iii) the coordination of the ester group in 1c to generate 1 G , this step being endergonic by 1.8 kcal/mol (Fig. 7 ; gray). Thus, the ester group participation for the replacement of N 2 in 1 A is not necessary. Next, a suprafacial α-aryl migration from Pd to the C≡C bond of 1 B ( syn -insertion) proceeds through transition state 1 TS α BC , found at 6.3 kcal/mol on the free energy surface, and results in the Pd- alkenyl ester complex 1 C α . This complex lies at –19.1 kcal/mol on the free energy surface with trans -relationship of two phenyl groups. Intramolecular neighboring group participation of the ester group at C α of 1 B can provide the Pd-alkenyl heterocyclic complex 1 D through 1 TS BD (12.6 kcal/mol); however, this process needs an additional 6.3 kcal/mol activation energy and is thus ruled out. Fig. 7 DFT calculations (atom colors: blue = Pd; yellow = S; red = O; gray = C; white = H). Full size image Alternatively, α-aryl migration of ester chelate 1 E forms intermediate 1 F α (–14.3 kcal/mol) through 1 TS α EF (10.7 kcal/mol). The energy barrier is 4.4 kcal/mol higher than 1 TS α BC ; this pathway is thus not preferred. A detailed comparison of all the options justifies the feasibility of the bottom pathway 1 B \({{\to }}\) 1 C α (marked in blue). Like normal Suzuki reactions, transmetalation of 1 C with aryl boronic acid followed by reductive elimination gives the final diarylation product (Supplementary Scheme 9 ). We have studied various tether lengths of the yne-acetate and found that the C α -arylation process is always favored over the C α -arylation (Supplementary Schemes 10 – 15 ). To rationalize this selectivity, a distortion/interaction and non-covalent interactions analysis of the aryl migration transition states 1 TS α BC and 1 TS β BC (that includes substrate fragment and aryl-palladium fragment) was performed (see right side in Fig. 7 and Supplementary Figs. 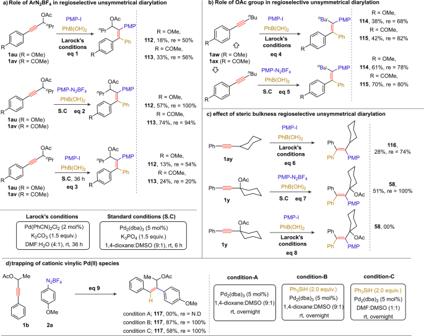Fig. 6: Mechanistic studies. aThree comparative reactions were performed with electronically diverse propargyl acetates under the {Larock’s reaction conditions: eq 1 [PMP-I, PhB(OH)2, Pd(PhCN)2Cl2, K2CO3, DMF:H2O (4:1), rt]}, {standard conditions (SC) of current reaction: eq 2 [PMP-N2BF4, PhB(OH)2, Pd2(dba)3, K3PO4, 1,4-dioxane:DMSO (9:1), rt]}, and {SC of current reaction: eq 3 [PMP-I instead of PMP-N2BF4]}. Excellent regioselectivity has been observed in eq 2; thus, PMP-N2BF4and cationic palladium species are pivotal.bTwo comparative reactions were performed with electronically diverse aryl-butyl alkynes using Larock’s reaction conditions (eq 4) and the SC of current reaction (eq 5).cTwo comparative reactions were independently performed with sterically hindered Ph-cyclohexyl alkyne and cyclohexyl tethered PA under the Larock’s reaction conditions (eqs. 6 and 8) and SC current reaction (eq. 7), respectively.dTrapping of cationic vinylic Pd(II) species in the absence of aryl boronic acid. Note: inseparable regioisomers are isolated as mixture and the regioisomeric excess (re) is determined by1H NMR. PMPp-methoxyphenyl. 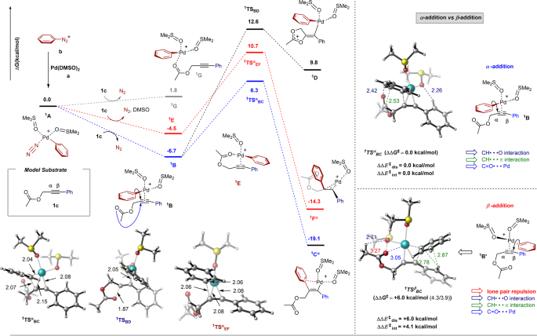Fig. 7 DFT calculations (atom colors: blue = Pd; yellow = S; red = O; gray = C; white = H). 14 – 16 ). The large rotation angle for β-aryl migration (see the SI: 36.12° for 1 TS β BC and 7.34° for 1 TS α BC ) contributes to excess distortion energy [+6.0 kcal/mol; that includes both aryl - palladium (+3.68 kcal/mol) and substrate (+2.32 kcal/mol) distortion]. In addition, a large level of non-covalent lone pair repulsion of the carboxylate moiety with ligated DMSO for 1 TS β BC (+4.1 kcal/mol) relative to 1 TS α BC was detected. In summary, a regio- and stereoselective syn -1,2-dicarbofunctionalization of unsymmetrical alkynes involving structurally distinct carbon functionalities has been developed. The cationic Pd II ‐catalyst plays an essential role in modulating the regioselective insertion of aryl‐diazonium salts and boronic acids/olefins to the unsymmetrical alkynes. The transformation proceeds at room temperature and tolerates oxidizable halo‐species (I/Br), easily transformable functionalities (CO 2 Me, CN) and strained rings, thus opening a broad chemical space [94 examples]. It is even successful on the gram scale. Carboxylate protecting group and the in situ formation of a stabilized cationic Pd intermediate solely responsible for the outcome and regioselectivity of syn -1,2-diarylation of unsymmetrical alkynes. DFT studies rationalize the α-arylation preference over β-arylation of PAs and discard direct participation of the acetate as a DG. The highly substituted olefins are subsequently used for the construction of functionalized indene, methyl-vinyl ketone, and acrolein skeletons. The current finding paves the way to the discovery of unknown difunctionalization strategies of unactivated alkynes. General procedure for the syn -1,2-difunctionalization reactions To a mixture of alkyne 1 (0.3 mmol), aryl diazonium tetrafluoroborate 2 (0.9 mmol), aryl boronic acid 3 or olefin 72 (0.45 mmol), Pd catalyst (0.015 mmol) and base (0.45 mmol) was added the respective solvent. The resulting reaction mixture was stirred at 25 °C for 6 h. The reaction progress was periodically monitored by TLC. The solvent was next removed either by water workup or by evaporation under reduced pressure. The organic layer was extracted in ethyl acetate (3 × 10 mL) and dried over Na 2 SO 4 . The organic layer was evaporated and purified by column chromatography over neutral alumina to afford 4 – 100 and 112 – 113 . The compounds are sensitive to acidic silica gel and thus, final product purification was carried out on neutral alumina.